The histone H2A deubiquitinase Usp16 regulates embryonic stem cell gene expression and lineage commitment Polycomb Repressive Complex 1 and histone H2A ubiquitination (ubH2A) contribute to embryonic stem cell (ESC) pluripotency by repressing lineage-specific gene expression. However, whether active deubiquitination co-regulates ubH2A levels in ESCs and during differentiation is not known. Here we report that Usp16, a histone H2A deubiquitinase, regulates H2A deubiquitination and gene expression in ESCs, and importantly, is required for ESC differentiation. Usp16 knockout is embryonic lethal in mice, but does not affect ESC viability or identity. Usp16 binds to the promoter regions of a large number of genes in ESCs, and Usp16 binding is inversely correlated with ubH2A levels, and positively correlates with gene expression levels. Intriguingly, Usp16 −/− ESCs fail to differentiate due to ubH2A-mediated repression of lineage-specific genes. Finally, Usp16, but not a catalytically inactive mutant, rescues the differentiation defects of Usp16 −/− ESCs. Therefore, this study identifies Usp16 and H2A deubiquitination as critical regulators of ESC gene expression and differentiation. Embryonic stem cells (ESCs) have the unique ability to differentiate into all somatic cell types [1] . This developmental plasticity is conferred by the pluripotent gene expression programme, which is maintained through a combination of ESC-specific transcription factors and recently characterized epigenetic regulators [2] , [3] , [4] . Polycomb group proteins are important epigenetic regulators that repress the expression of key developmental regulators in ESCs, thus stabilizing the pluripotent gene expression programme [3] , [5] , [6] . Two major Polycomb repressive complexes (PRCs), designated as PRC1 and PRC2, have been described. PRC2 mediates di- and tri-methylation of histone H3 lysine 27 (H3K27me2/3) [7] , [8] , [9] , [10] , while PRC1 subunits Ring1A/B catalyse ubiquitination of histone H2A lysine 119 (ubH2A) [11] , [12] . Interestingly, some genes enriched for H3K27me2/3 are also enriched for H3K4me3, a mark generally found at actively transcribed genes [13] . These bivalent modifications are found principally at key developmental regulators and may help repress these genes in ESCs while enabling their rapid induction in response to developmental signals [14] . Recent investigations reveal that PRC1-mediated ubH2A also marks bivalent genes and regulates their expression in ESCs [15] , [16] , [17] . Simultaneous depletion of Ring1A and Ring1B in ESCs causes de-repression of bivalent genes and loss of ESC identity [16] , [18] . Therefore, PRC1 binding and, possibly, PRC1-mediated H2A ubiquitination, may be required for the efficient repression of key development-related genes in ESCs. Interestingly, recent studies reveal that ubH2A is enriched at promoters of genes involved in metabolism and other processes, suggesting additional roles for Ring1B and ubH2A in ESCs [19] . Reinforcing the links between Ring1B, ubH2A and transcriptional silencing, genes bound by PRC1 and enriched for ubH2A in ESCs are associated with RNAPII-S5P, which does not produce mature mRNA [19] . This is consistent with a role for ubH2A in transcriptional repression [18] , [19] , [20] , [21] . However, non-enzymatic PRC1 function may also contribute to gene repression by directly compacting chromatin, blocking remodelling, inhibiting transcription initiation and repressing gene expression [22] , [23] , [24] , [25] . Unambiguously demonstrating the functions of ubH2A in PRC1-mediated gene repression in vivo remains a challenge in higher eukaryotes. Like other histone modifications, ubH2A is a reversible mark that is removed through the activity of deubiquitinating enzymes. The levels of cellular ubH2A are determined by the balance between PRC1-mediated ubH2A and ubH2A deubiquitination. A number of ubH2A deubiquitinases have been reported, including USP16 (Ubp-M), 2A-DUB (MYSM1), USP21, USP7, USP3 and Drosophila calypso [26] , [27] , [28] , [29] , [30] . Interestingly, USP16, which is located on human chromosome 21 and triplicated in Down’s syndrome, reduces the self-renewal of hematopoietic stem cells and the expansion of mammary epithelial cells, neural progenitors and fibroblasts in mice, suggesting that Usp16 may antagonize PRC1 function in the self-renewal and/or senescence pathways [31] . Usp16 has also been shown to coordinate with Aurora B-mediated H3S28 phosphorylation to facilitate transcription in quiescent lymphocytes [32] . However, the specific enzyme that reverses PRC1-mediated H2A ubiquitination in ESCs to regulate ubH2A levels is not known. During ESC differentiation, bivalent histone modifications are resolved to monovalent modifications [14] and pluripotency-specific genes are epigenetically silenced [33] , [34] . However, the mechanisms by which repressive H3K27me and ubH2A marks are resolved remain largely unknown. Two JmjC-domain-containing proteins, UTX and JMJD3, can actively remove H3K27me and, therefore, may counteract PRC2-mediated gene silencing during ESC differentiation [35] , [36] . Although, there are several known histone H2A deubiquitinases, none have yet been linked to ESC differentiation [26] , [27] , [28] , [29] , [30] . Whether ubH2A deubiquitination is important during ESC differentiation and which enzyme mediates ubH2A deubiquitination during cell fate transitions is not known. In this study, we report that Usp16 regulates H2A deubiquitination and gene expression in mouse ESCs and during ESC differentiation. Although Usp16 −/− ESCs are viable and exhibit normal morphology, gene expression and ubH2A profiles are altered. We further demonstrate that Usp16-mediated ubH2A deubiquitination is essential for ESC differentiation. Usp16 −/− ESCs fail to activate lineage-specific gene expression and undergo lineage commitment due to the inability of these cells to remove the repressive ubH2A mark at key developmental regulators. Finally, we demonstrate that Usp16, but not the enzymatically inactive mutant, rescues the differentiation defects of Usp16 −/− ESCs. Therefore, this study demonstrates that Usp16 regulates H2A deubiquitination and gene expression in ESCs and Usp16-mediated H2A deubiquitination plays critical roles during ESC differentiation. Usp16 knockout is early embryonic lethal in mice USP16 was first identified as a histone H2A-specific deubiquitinase that regulates cell cycle progression and gene expression in human cells [26] . To determine whether Usp16 is essential for mammalian development, we knocked out the gene in murine ESCs and produced mice. The targeting vector was designed to replace exons 5 and 6 of mouse Usp16 with a PGK-Neo/Kan cassette ( Fig. 1a ). Cysteine 205 in exon 6 is required for Usp16 deubiquitinase activity ( Fig. 1a ). The targeting vector was electroporated into the F1 hybrid (B6/129) ESC line V6.5 and G418 resistant colonies were selected ( Fig. 1a ). After removing the PGK-Neo/Kan cassette by transient expression of Cre-recombinase, correctly targeted ESCs were identified by PCR-mediated genotyping ( Fig. 1b ) and injected into blastocysts to produce mice. After germline transmission, mice heterozygous for Usp16 deletion (Usp16 +/− ) were inbred to obtain Usp16 knockout mice (Usp16 −/− ). However, no homozygous Usp16 knockout mice were obtained ( Fig. 1c , 89 mice, 12 litters), indicating that Usp16 deletion is embryonic lethal. 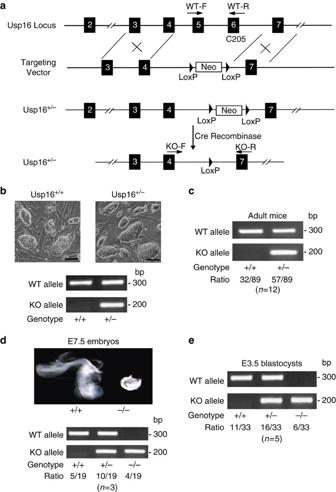Figure 1: Usp16 is required for mouse embryonic development. (a) Schematic representation of the strategies used to generate Usp16 knockout mice. Partial regions of Usp16 locus (from exons 2 to 7) are shown. Exons are shown as filled boxes and LoxP sites as filled triangles. PCR primers used for genotyping are shown as arrows. Position of cysteine 205, an amino acid essential for Usp16 deubiquitination activity, is indicated. (b) Identification of correctly targeted mouse embryonic stem cells. Top panels, phase contrast of the morphology of correctly targeted Usp16 ESCs as compared with wild-type V6.5 ESCs. Bottom panel, images of genotyping results of ESCs as shown in the top panel. PCR reactions were performed using primers as indicated in panel A. Scale bar, 50 μm. (c) Usp16 is required for mouse viability. Images of PCR genotyping of offspring from Usp16+/−mice intercrossing. The number and ratio of wild type and heterozygote adult mice genotyped were shown (the number in the parenthesis indicates litters examined). (d) Usp16 knockout results in early embryonic lethal. Image and PCR genotyping of E7.5 embryos from Usp16+/−mice intercrossing showing partially re-absorption of Usp16−/−embryos. The number and ratio of embryos genotyped were shown (the number in the parenthesis indicates litters examined). (e) Usp16−/−blastocysts are viable. PCR genotyping of blastocysts from Usp16+/−intercrossing. The number and ratio of blastocysts genotyped were shown under the PCR image (the number in the parenthesis indicates female mice killed). Original scans for gels are shown inSupplementary Fig. 7. Figure 1: Usp16 is required for mouse embryonic development. ( a ) Schematic representation of the strategies used to generate Usp16 knockout mice. Partial regions of Usp16 locus (from exons 2 to 7) are shown. Exons are shown as filled boxes and LoxP sites as filled triangles. PCR primers used for genotyping are shown as arrows. Position of cysteine 205, an amino acid essential for Usp16 deubiquitination activity, is indicated. ( b ) Identification of correctly targeted mouse embryonic stem cells. Top panels, phase contrast of the morphology of correctly targeted Usp16 ESCs as compared with wild-type V6.5 ESCs. Bottom panel, images of genotyping results of ESCs as shown in the top panel. PCR reactions were performed using primers as indicated in panel A. Scale bar, 50 μm. ( c ) Usp16 is required for mouse viability. Images of PCR genotyping of offspring from Usp16 +/− mice intercrossing. The number and ratio of wild type and heterozygote adult mice genotyped were shown (the number in the parenthesis indicates litters examined). ( d ) Usp16 knockout results in early embryonic lethal. Image and PCR genotyping of E7.5 embryos from Usp16 +/− mice intercrossing showing partially re-absorption of Usp16 −/− embryos. The number and ratio of embryos genotyped were shown (the number in the parenthesis indicates litters examined). ( e ) Usp16 −/− blastocysts are viable. PCR genotyping of blastocysts from Usp16 +/− intercrossing. The number and ratio of blastocysts genotyped were shown under the PCR image (the number in the parenthesis indicates female mice killed). Original scans for gels are shown in Supplementary Fig. 7 . Full size image To determine the stage at which Usp16 deletion is lethal, Usp16 +/− male and female mice were mated and embryos were isolated. No Usp16 −/− embryos were detected at embryonic day (E) 13.5 or E10.5. However, Usp16 −/− embryos were detected at E7.5. The majority of E7.5 embryos displayed normal morphology, with closed neural tubes ( Fig. 1d ). In contrast, a small number of embryos appeared to be partially re-absorbed ( Fig. 1d ). Morphologically normal embryos were either Usp16 +/+ or Usp16 +/− while the partially re-absorbed embryos were Usp16 −/− ( Fig. 1d ). These results indicate that defects in Usp16 −/− embryos occurred before E7.5. To determine whether Usp16 deletion affects embryo viability before or after implantation, we collected blastocysts at E3.5. Genotyping analysis of 33 blastocysts recovered from 5 female mice identified 6 Usp16 −/− embryos ( Fig. 1e ). This result indicates that Usp16 knockout causes lethal developmental defects after implantation but before the E7.5 developmental stage. Usp16 knockout does not affect ESC viability and identity Similar to Usp16 deletion, knockout of any of the PRC subunits in mice, such as Suz12, Ezh2, Eed or Ring1B, results in early embryonic lethality [37] , [38] , [39] , [40] . ESCs deficient for these PRC subunits are viable, but are prone to spontaneously differentiate during culture. Therefore, we reasoned that Usp16 knockout ESCs should also be viable. To study the role of Usp16 in early mouse embryonic development, we first derived Usp16 −/− ESCs by culturing blastocysts in 2i medium. Surprisingly, of 45 ESC lines derived by this method, 17 were Usp16 +/+ , 28 were Usp16 +/− and none were Usp16 −/− . The successful generation of multiple Usp16 +/+ and Usp16 +/− ESC lines suggests that our inability to generate Usp16 −/− ESC lines was not due to technical reasons. One possible explanation is that Usp16 is required for gene expression reprogramming during the blastocyst to ESCs transition. To test this hypothesis, we derived Usp16 −/− ESCs by targeting the remaining wild-type allele in the Usp16 +/− ESCs, which were used to generate Usp16 knockout mice. For this purpose, we constructed a conditional targeting vector by inserting a LoxP site upstream of exon 5 and a PGK-Neo/Kan cassette (which was flanked with two FRT sites and one downstream LoxP site) downstream of Usp16 exon 6 ( Supplementary Fig. 1a ). This vector was then electroporated into the Usp16 +/− ESCs to replace the remaining wild-type Usp16 allele. Since the homologous regions of the conditional targeting vector have been deleted in the Usp16 knockout allele, the wild-type allele should be specifically replaced. ESCs in which the remaining wild-type allele was replaced were selected by G418 resistance. The PGK-Neo/Kan cassette was then removed by transient expression of Flippase and used for the generation of Usp16 conditional knockout mice ( Supplementary Fig. 1a ; see below). Usp16 was deleted from these ESCs by transient expression of Cre recombinase ( Supplementary Fig. 1a ). Usp16 −/− ESCs were identified by PCR-mediated genotyping ( Supplementary Fig. 1c ) and confirmed by western blot and real-time PCR analysis ( Supplementary Fig. 1d ; Supplementary Fig. 1e ). Usp16 −/− ESCs exhibited normal morphology ( Supplementary Fig. 1b ) and expressed pluripotent genes at levels similar to control V6.5 ESCs ( Supplementary Fig. 1e ). Therefore, even though direct derivation of Usp16 −/− ESCs from blastocysts could not be achieved, Usp16 does not appear to be required for ESC viability. Since Usp16 −/− ESCs generated by the above-described approach have been subjected to multiple rounds of electroporation, which might alter cellular functions, we also derived Usp16 −/− ESCs by an alternative approach. We took advantage of Usp16 conditional knockout mice, which were generated by injecting Usp16 2Lox ESCs ( Supplementary Fig. 1a ) into blastocysts (data not published). These conditional Usp16 knockout (Usp16 2lox/2lox ) mice were crossed with the inducible Cre expression mouse line, CAGG-Cre, to obtain Usp16 2lox/+ : CAGG-Cre mice. These mice were then interbred or bred with Usp16 2lox/2lox mice. ESCs were derived from the offspring of these crossings and Usp16 2lox/2lox :CAGG-Cre ESCs were identified by PCR-mediated genotyping and confirmed by sequencing ( Fig. 2a ). Usp16 was deleted by culturing Usp16 2lox/2lox :CAGG-Cre ESCs with 1 μM 4-hydroxytamoxifen (4-OHT), which induces nuclear localization of the Cre recombinase, for 3–5 days ( Fig. 2a ) before switching to 4-OHT free medium. The efficiency of Usp16 deletion was confirmed by western blot assay ( Fig. 2c ). Consistent with our previous studies, Usp16 knockout caused a specific increase of ubH2A levels, but had no effect on ubH2B levels ( Fig. 2c , the intensity of ubH2A signal were quantified and labelled). Usp16 −/− ESCs exhibited normal morphology ( Fig. 2b ) and have growth rates ( Fig. 2e ) and cell cycle profiles ( Fig. 2f ) similar to Usp16 +/+ ESCs. This contrasts with studies in HeLa cells, where USP16 deletion causes a slow growth phenotype, partially due to the defects of H2A deubiquitination during cell cycle G2/M phase progression [26] , [41] . Usp16 −/− ESCs stained positively for alkaline phosphatase ( Fig. 2b ). Pluripotent genes Oct4, Sox2 and Nanog and PRC subunits Ring1B, Suz12 and Ezh2 were not affected by Usp16 deletion ( Fig. 2d ). Together, these studies demonstrate that Usp16 regulates ubH2A levels in ESCs, and is not required for ESC viability and identity. 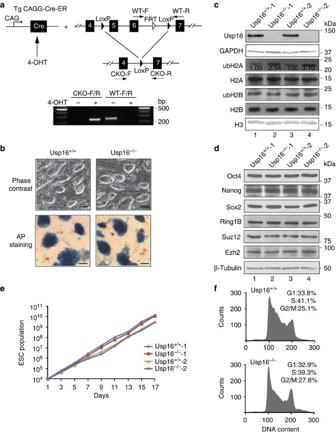Figure 2: Usp16 knockout does not affect ESC viability and identity. (a) Schematic representation of the strategy used to delete Usp16 (top panels) and an image of genotyping result of Usp16 deleted ESCs (bottom panel). PCR primers used for genotyping are indicated in the top panel. (b) Phase-contrast images (top panels) and alkaline phosphatase staining images (bottom panels) of Usp16+/+and Usp16−/−ESCs. Scale bar, 50 μm. (c) Western blot analysis of Usp16 (top panel), H2A ubiquitination (third panel) and H2B ubiquitination (fifth panel) levels in two independent Usp16+/+and Usp16−/−ESC lines. The quantification of ubH2A signals was labelled. Signals in control Usp16+/+ESCs were arbitrarily set as 1. GAPDH, histone H2A, H2B and H3 were used as loading controls. (d) Western blot analysis of the levels of pluripotent genes and PRC subunits in two independent control Usp16+/+and Usp16−/−ESC lines. β-tubulin was used as a loading control. (e) Growth curve of two independent control Usp16+/+and Usp16−/−ESC lines. A total of 1 × 104ESCs were seeded in 12-well plates and cell numbers were counted every other day. The same seeding procedure was repeated every other day. (f) Fluorescence-activated cell sorting (FACS) analysis of control Usp16+/+and Usp16−/−ESC lines. The percentages of cell populations at each cell cycle phase were labelled. Original scans for gels and blots are shown inSupplementary Fig. 7. Figure 2: Usp16 knockout does not affect ESC viability and identity. ( a ) Schematic representation of the strategy used to delete Usp16 (top panels) and an image of genotyping result of Usp16 deleted ESCs (bottom panel). PCR primers used for genotyping are indicated in the top panel. ( b ) Phase-contrast images (top panels) and alkaline phosphatase staining images (bottom panels) of Usp16 +/+ and Usp16 −/− ESCs. Scale bar, 50 μm. ( c ) Western blot analysis of Usp16 (top panel), H2A ubiquitination (third panel) and H2B ubiquitination (fifth panel) levels in two independent Usp16 +/+ and Usp16 −/− ESC lines. The quantification of ubH2A signals was labelled. Signals in control Usp16 +/+ ESCs were arbitrarily set as 1. GAPDH, histone H2A, H2B and H3 were used as loading controls. ( d ) Western blot analysis of the levels of pluripotent genes and PRC subunits in two independent control Usp16 +/+ and Usp16 −/− ESC lines. β-tubulin was used as a loading control. ( e ) Growth curve of two independent control Usp16 +/+ and Usp16 −/− ESC lines. A total of 1 × 10 4 ESCs were seeded in 12-well plates and cell numbers were counted every other day. The same seeding procedure was repeated every other day. ( f ) Fluorescence-activated cell sorting (FACS) analysis of control Usp16 +/+ and Usp16 −/− ESC lines. The percentages of cell populations at each cell cycle phase were labelled. Original scans for gels and blots are shown in Supplementary Fig. 7 . Full size image Usp16 binding with relation to gene expression and ubH2A level Since Usp16 regulates ubH2A levels in ESCs, and PRC1 and H2A ubiquitination are enriched at developmental and metabolic genes in ESCs [15] , [19] , we investigated whether Usp16 regulates gene expression in ESCs by RNA-sequencing (RNA-seq). Usp16 knockout was associated with an apparent decrease of transcript abundance ( Supplementary Fig. 2a ), consistent with the role of Usp16 as a histone H2A deubiquitinase functioning in gene activation. A total of 1,094 genes were significantly differentially expressed (Log 2 [Fold change] >2 cutoff), with 330 genes upregulated and 764 genes downregulated in Usp16 −/− ESCs ( Fig. 3a ). Upregulated genes are particularly enriched for myofibril assembly, macromolecular complex assembly, chromatin assembly and nucleosome organization, while downregulated genes are enriched for transcription regulation, RNA, nitrogen and macromolecule metabolism ( Supplementary Fig. 2b ), indicating that further increasing ubH2A levels by inactivation of Usp16 affects many basic cellular processes However, removing ubH2A by knocking out Ring1A/1B and further increasing ubH2A by inactivation of Usp16 primarily affect distinct groups of genes, only 12.6% of Usp16 knockout affected genes (1,094, including both up- and downregulated, Fig. 3a ) overlaps with genes affected by Ring1A/B inactivation (1,156, including both up- and downregulated) [18] ( Supplementary Fig. 2d ). Since Usp16 knockout ESCs maintain ESC identity, the deregulation of these genes does not appear to impede ESC self-renewal. However, USP16 −/− ESCs do have a higher tendency for differentiation under certain culture conditions compared with Usp16 +/+ ES cells ( Supplementary Fig. 2e ), indicating that Usp16-regulated gene expression also contributes to the stabilization of the pluripotent gene expression programme. We further validated the RNA-seq results by real-time PCR of 10 randomly selected genes ( Supplementary Fig. 2c ). These results confirmed our RNA-seq data and revealed that Usp16 regulates gene expression in ESCs. 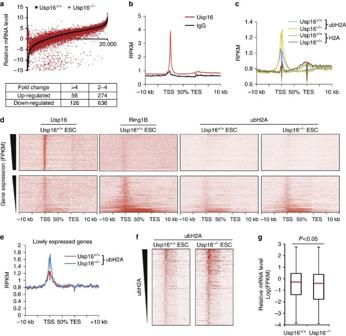Figure 3: Usp16 binds to TSS and positively correlates with gene expression and inversely correlates with H2A deubiquitination levels. (a) Scatter plot of gene expression levels in Usp16+/+and Usp16−/−ESCs as determined by RNA-seq. The fragments per kilobase of exon model per million mapped reads (FPKM) was calculated for each transcript using Cufflinks and transformed to Log2 (FPKM) as relative RNA level. Genes that are significantly deregulated (Log2[Fold change]>2) in Usp16−/−ESCs were shown in the bottom table. (b) Binding of Usp16 (red line) and IgG (black line) to gene-coding regions plus 10 kb upstream of the TSS and downstream of transcription ending site (TES) in Usp16+/+ESCs. Parallel experiments in Usp16−/−ESCs were shown inSupplementary Fig. 3c. (c) ubH2A (orange line, Usp16−/−; blue line, Usp16+/+) and H2A (brown line, Usp16−/−; green line, Usp16+/+) signals across gene-transcribing regions plus 10 kb upstream of TSS and downstream of TES. (d) Usp16 (first column), Ring1B (second column) and ubH2A (third and fourth columns) distribution at individual genes in Usp16+/+and Usp16−/−ESCs. Top row, top 1,000 expressed genes sorted by relative expression (FPKM). Bottom row, bottom 1,000 expressed genes in gene list re-sorted based on Ring1B signal. Analyses span 10 kb upstream of the TSS, the gene body, and 10 kb downstream of the TES. (e) Binding profiles of ubH2A in bottom 1,000 expressed genes re-sorted by Ring1B binding in Usp16+/+and Usp16−/−ESCs. (f) ubH2A distribution at individual genes in Usp16+/+and Usp16−/−ESCs. Genes are sorted based on ubH2A signals in Usp16+/+ESCs. (g) Expression levels of genes infin Usp16+/+and Usp16−/−ESCs.P-value is calculated by the Student’st-test. Top whisker and bar represent 98th percentile of genes. Bottom whisker and bar represent 2nd percentile of genes above zero. Figure 3: Usp16 binds to TSS and positively correlates with gene expression and inversely correlates with H2A deubiquitination levels. ( a ) Scatter plot of gene expression levels in Usp16 +/+ and Usp16 −/− ESCs as determined by RNA-seq. The fragments per kilobase of exon model per million mapped reads (FPKM) was calculated for each transcript using Cufflinks and transformed to Log2 (FPKM) as relative RNA level. Genes that are significantly deregulated (Log 2 [Fold change]>2) in Usp16 −/− ESCs were shown in the bottom table. ( b ) Binding of Usp16 (red line) and IgG (black line) to gene-coding regions plus 10 kb upstream of the TSS and downstream of transcription ending site (TES) in Usp16 +/+ ESCs. Parallel experiments in Usp16 −/− ESCs were shown in Supplementary Fig. 3c . ( c ) ubH2A (orange line, Usp16 −/− ; blue line, Usp16 +/+ ) and H2A (brown line, Usp16 −/− ; green line, Usp16 +/+ ) signals across gene-transcribing regions plus 10 kb upstream of TSS and downstream of TES. ( d ) Usp16 (first column), Ring1B (second column) and ubH2A (third and fourth columns) distribution at individual genes in Usp16 +/+ and Usp16 −/− ESCs. Top row, top 1,000 expressed genes sorted by relative expression (FPKM). Bottom row, bottom 1,000 expressed genes in gene list re-sorted based on Ring1B signal. Analyses span 10 kb upstream of the TSS, the gene body, and 10 kb downstream of the TES. ( e ) Binding profiles of ubH2A in bottom 1,000 expressed genes re-sorted by Ring1B binding in Usp16 +/+ and Usp16 −/− ESCs. ( f ) ubH2A distribution at individual genes in Usp16 +/+ and Usp16 −/− ESCs. Genes are sorted based on ubH2A signals in Usp16 +/+ ESCs. ( g ) Expression levels of genes in f in Usp16 +/+ and Usp16 −/− ESCs. P -value is calculated by the Student’s t -test. Top whisker and bar represent 98th percentile of genes. Bottom whisker and bar represent 2nd percentile of genes above zero. Full size image To determine whether Usp16 regulates H2A ubiquitination level at PRC1 target genes in ESCs, we first determined the Usp16-binding profile in ESCs by ChIP sequencing (ChIP-seq). ChIP-sequencing results revealed that USP16 binds to all chromosomes with no particular bias for any individual chromosomes ( Supplementary Fig. 3a ). Tag counts normalized to the coverage of different gene structures revealed that USP16 binding is particularly enriched in the proximal regions (2 kb upstream) of transcription start site (TSS) and 5′UTR with relatively low strength in 5′ distal regions (50 kb upstream of TSS), gene-coding regions (both exons and introns), 3′ UTR, 2 kb downstream of TTS, 3 distal region (50 kb) and non-genic regions compared with IgG ( Supplementary Fig. 3b ). To gain insight into the role of Usp16 in gene regulation, we performed a metagene analysis combining all genes in the mouse genome, including up and downstream regions. This analysis revealed that USP16 specifically binds to gene promoter regions, defined as −2 kb to +1 kb of TSS sites ( Fig. 3b ). Parallel ChIP-seq experiments with Usp16 antibody in Usp16 −/− ESCs did not reveal any significant binding ( Supplementary Fig. 3c ), indicating the specificity of ChIP-seq signals. To better understand the significance of Usp16 binding, we employed peak calling analysis (see Methods) and identified ~7,000 Usp16-binding sites, which occupy 4,814 promoters. Usp16-bound genes are enriched for genes encoding proteins involved in RNA processing, RNA binding, protein localization, macromolecule catabolic process, protein transport, DNA binding, cell cycle, chromosome organization, protein biosynthesis, DNA repair, RNA polymerase activity and proteasome complex, indicating a potential and wide-spread function of Usp16 in regulating a variety of fundamental cellular processes, although only limited amounts of genes show significant changes when Usp16 is inactivated ( Supplementary Fig. 3d ). To determine the site-specific effects of Usp16 on H2A ubiquitination, we measured ubH2A levels in Usp16 +/+ and Usp16 −/− ESCs by native ChIP-seq. Consistent with recent studies, ubH2A was enriched at gene promoters ( Fig. 3c ) [19] , [21] . By using peak calling analysis, we identified 2,433 gene promoters significantly enriched for ubH2A. These genes strongly overlap with ubH2A enriched genes reported in a recent study (75% overlapping, similar binding profiles and similar GO categories; Supplementary Fig. 3e ) [19] , indicating the reliability of our native ChIP-seq experiments. Genes bound by ubH2A are mainly developmental and transcription regulators ( Supplementary Fig. 4a ). A total of 2,022 genes become newly enriched for ubH2A in Usp16 −/− ESCs, indicating a significant role for Usp16 in regulating ubH2A levels at these genes ( Supplementary Fig. 4a ). These genes include some developmental regulators but are mainly enriched for general biological processes, consistent with recent report [19] ( Supplementary Fig. 4a ). Supporting our biochemical assays, Usp16 knockout caused a significant increase of ubH2A levels without any apparent effects on H2A levels ( Fig. 3c ). To better define the relationships between Usp16, ubH2A level, PRC1 and gene expression on a gene-by-gene basis we generated binding profile heat maps. Genes were sorted based on expression level ( Fig. 3d ; the 1,000 highest and least expressed genes are shown). Since the bottom genes are largely unexpressed (FPKM<1), we re-sorted these genes using Ring1B binding extracted from a recent publication [42] . The heatmaps of Usp16 binding reinforces the metagene analysis, illustrating localization specific to the promoter regions of virtually all genes ( Fig. 3d ). Furthermore, consistent with a role in promoting transcriptional activity, Usp16 was more highly enriched at active promoters than silent genes ( Fig. 3d ). Ring1B localization was also specific to the promoter regions of virtually all genes, but its binding was more prominent among the silent genes than in the most highly expressed ( Fig. 3d ). Consistent with each protein’s enzymatic activity, ubH2A was virtually undetectable at active genes (where Usp16 was most abundant), and accumulated among silent genes (where Ring1B was most abundant) ( Fig. 3d ). Furthermore, the heatmaps clearly illustrate the strong correlation between the presence of Ring1B and that of ubH2A, as previously reported [15] , [19] , [21] . Both the heatmap and metagene analysis illustrate that ubH2A levels are markedly increased in Usp16 −/− ESCs ( Fig. 3d–f , Supplementary Fig. 4c ). Visualization of H2A signal did not reveal changes in H2A signal in Usp16 +/+ or Usp16 −/− ESCs ( Supplementary Fig. 4b ), indicating the specificity of the detected ubH2A changes. Further evidence that Usp16 and Ring1B competitively regulate ubH2A levels was provided by conventional ChIP-qPCR assay. As shown in Supplementary Fig. 4d , overexpression of Ring1B and Usp16 increased the levels of these proteins at gene promoters. Importantly, overexpression of Ring1B correlates with an increase of ubH2A and overexpression of Usp16 correlates with a decrease of ubH2A at gene promoters ( Supplementary Fig. 4d ). Consistent with a role of ubH2A in gene repression, ubH2A-enriched genes have decreased expression in response to Usp16 knockout ( Fig. 3g ). In summary, these data reveal that Usp16 binds to gene promoter, positively correlates with gene expression and inversely correlates with Ring1B binding and H2A ubiquitination levels. Usp16 −/− ESCs are defective for differentiation Although Usp16 is not required for ESC identity, Usp16 knockout is lethal during early embryogenesis in mice, suggesting that Usp16 knockout may affect ESC differentiation. To determine whether Usp16 regulates ESC differentiation, we differentiated Usp16 −/− and Usp16 +/+ ESCs by forming embryoid bodies (EBs) and compared their phenotypes. The number of EBs formed from Usp16 −/− ESCs (Usp16 −/− EBs) is similar to the number of Usp16 +/+ ESC derived EBs (Usp16 +/+ EBs), indicating that Usp16 knockout does not affect EB formation ( Supplementary Fig. 4e ; data not shown). The morphology of Usp16 +/+ EBs was heterogeneous and contained multiple condensed regions refractory to light ( Fig. 4a ). In contrast, Usp16 −/− EBs were more homogeneous, containing fewer light refractory regions and a smaller condensed central region ( Fig. 4a ). The transparency difference indicates that, even though both ESCs can form EBs, the internal structure of Usp16 −/− and Usp16 +/+ EBs differ. In addition, Usp16 −/− EBs exhibited a distinct growth curve ( Fig. 4b ). Usp16 +/+ EBs grew rapidly, showing a dramatic increase in diameter between day 3 and day 7 before reaching a plateau between days 7–8. In contrast, Usp16 −/− EBs grew more slowly, did not exhibit staged growth and had not reached maximal growth by the end of the experiment (days 9–12). To better identify the differences between these EBs, we sectioned day 12 EBs and analysed them by haematoxylin and eosin staining. As shown in Fig. 4c , Usp16 +/+ EBs exhibited heterogeneous staining and showed different germ layer morphology, such as small cavity structures. In contrast, Usp16 −/− EBs stained more homogenously and contained undifferentiated cell clumps, with central regions of dead and apoptotic cells ( Fig. 4c ). These studies reveal that Usp16 −/− ESCs are unable to undergo normal differentiation. 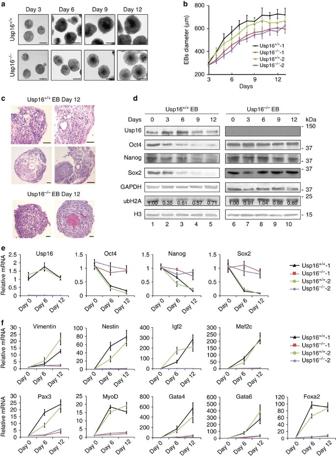Figure 4: Usp16−/−ESCs are defective for differentiation. (a) Phase-contrast images of EB morphology during EB formation from Usp16+/+and Usp16−/−ESCs. (b) Growth curve of EBs formed from Usp16+/+and Usp16−/−ESCs. The diameter of EBs at each day was measured and compared. For each time point, 50 EB diameters were measured. Means and s.d. (error bars) are shown. (c) Haematoxylin and eosin staining of day12 EBs formed from Usp16+/+and Usp16−/−ESCs. Day 12 EBs from Usp16−/−ESCs lack organized structure and failed to differentiate. Scale bar, 100 μm. (d) Western blot analysis of the levels of Usp16 (top panel), ubH2A (sixth panel) and pluripotent genes (second to fourth panels) during EB formation. ubH2A signals were quantified as inFig. 2c. Signals in Usp16+/+EBs at day 0 were arbitrarily set as 1. GAPDH and histone H3 were used as loading controls. Original scans for blots are shown inSupplementary Fig. 7. (e) Real-time PCR analysis of Usp16 and pluripotent genes expression at day 0, day 6 and day 12 during EB formation of two independent Usp16+/+and Usp16−/−ESC lines. Gene expression levels at day 0 were arbitrarily set as 1. Bars represent means+s.d. Number of biological replicatesn=3. (f) Real-time PCR analysis of lineage-specific genes expression at day 0, day 6 and day 12 during EB formation from two independent Usp16+/+and Usp16−/−ESC lines. Gene expression levels at day 0 were arbitrarily set as 1. Bars represent means+s.d. Number of biological replicatesn=3. Figure 4: Usp16 −/− ESCs are defective for differentiation. ( a ) Phase-contrast images of EB morphology during EB formation from Usp16 +/+ and Usp16 −/− ESCs. ( b ) Growth curve of EBs formed from Usp16 +/+ and Usp16 −/− ESCs. The diameter of EBs at each day was measured and compared. For each time point, 50 EB diameters were measured. Means and s.d. (error bars) are shown. ( c ) Haematoxylin and eosin staining of day12 EBs formed from Usp16 +/+ and Usp16 −/− ESCs. Day 12 EBs from Usp16 −/− ESCs lack organized structure and failed to differentiate. Scale bar, 100 μm. ( d ) Western blot analysis of the levels of Usp16 (top panel), ubH2A (sixth panel) and pluripotent genes (second to fourth panels) during EB formation. ubH2A signals were quantified as in Fig. 2c . Signals in Usp16 +/+ EBs at day 0 were arbitrarily set as 1. GAPDH and histone H3 were used as loading controls. Original scans for blots are shown in Supplementary Fig. 7 . ( e ) Real-time PCR analysis of Usp16 and pluripotent genes expression at day 0, day 6 and day 12 during EB formation of two independent Usp16 +/+ and Usp16 −/− ESC lines. Gene expression levels at day 0 were arbitrarily set as 1. Bars represent means+s.d. Number of biological replicates n =3. ( f ) Real-time PCR analysis of lineage-specific genes expression at day 0, day 6 and day 12 during EB formation from two independent Usp16 +/+ and Usp16 −/− ESC lines. Gene expression levels at day 0 were arbitrarily set as 1. Bars represent means+s.d. Number of biological replicates n =3. Full size image To determine whether the defects in Usp16 −/− ESC differentiation are linked to H2A ubiquitination, we analysed the levels of ubH2A, Usp16 and pluripotent gene markers during EB formation. Usp16 expression exhibits a dynamic change during EB formation, increasing at early stages of ESC differentiation, peaking at days 3–6 and then decreasing to ESC levels after day 6 ( Fig. 4d ). ubH2A levels during EB formation were largely inversely correlated with Usp16 levels and decreased during the initial stage of EB formation before gradually returning to the levels in ESCs ( Fig. 4d ; the intensity of ubH2A was measured and labelled). In contrast, Usp16 −/− EBs did not exhibit the same dynamic change of ubH2A levels ( Fig. 4d ). Moreover, while pluripotent genes Oct4, Nanog and Sox2 were quickly repressed in Usp16 +/+ EBs, becoming undetectable after day 6 ( Fig. 4d ), these genes remained at high levels in day 12 Usp16 −/− EBs ( Fig. 4d ). To further confirm the western blot results, we measured the RNA levels of pluripotent genes as well as markers for the three primary germ layers in day 6 and day 12 EBs by RT–qPCR assay. Consistent with the western blot results, the expression of Usp16 in Usp16 +/+ EBs at day 6 is higher than at both days 0 and 12. There is no detectable expression of pluripotent genes Oct4, Nanog and Sox2 at day 12 ( Fig. 4e ), but lineage-specific markers for ectoderm (Vimentin, Nestin and Igf2), mesoderm (Mef2c, Pax3 and MyoD) and endoderm (Gata4, Gata6 and Foxa2) are expressed at high levels ( Fig. 4f ). In contrast, Usp16 −/− EBs did not express these lineage-specific markers and maintained high expression levels of pluripotent genes even at day 12 ( Fig. 4e,f ). Taken together, these data reveal that Usp16 is required to activate cell type-specific gene expression programs and repress the expression of pluripotent markers during ESC differentiation. Usp16 is required for removing ubH2A mark during ESC differentiation PcG proteins regulate gene repression, at least in part, through covalent modification of histones [7] , [12] . During cell fate transitions, the repressive chromatin marks H3K27me and ubH2A are selectively resolved at bivalent genes to specify new, lineage-specific gene expression profiles. Our studies on EBs formed from Usp16 −/− ESCs suggest an intriguing working model wherein Usp16-mediated H2A deubiquitination relieves ubH2A-mediated repression to activate genes required for proper cell lineage commitment. Our studies revealed that Usp16 −/− ESCs fail to activate germ layer markers when stimulated to differentiate ( Fig. 4f ). To determine the effects of Usp16 deletion on gene expression during differentiation, we performed RNA-seq on day 12 EBs. In contrast to the relatively small numbers of differentially expressed genes in Usp16 −/− ESCs, 2,371 genes exhibited significant changes (Log 2 [Fold change] >2), with 785 genes upregulated and 1,586 genes downregulated ( Fig. 5a ). Gene ontology analysis revealed that the majority of downregulated genes are involved in development ( Supplementary Fig. 5a ). Genes upregulated are mainly related to metabolism, biosynthesis or early-stage developmental processes such as mesoderm development or blastocyst development ( Supplementary Fig. 5b ). This indicates that Usp16 is required for the normal ESC differentiation process. By comparing the gene expression profiles of Usp16 +/+ ESCs and EBs, we identified ~1,200 genes upregulated ( Fig. 5b ) and 700 genes downregulated during normal ESC differentiation ( Fig. 5b ). These differentially expressed genes reflect the normal reprogramming of the gene expression profile during ESC differentiation. Interestingly, the majority of these genes are misregulated during in vitro differentiation of Usp16 −/− ESCs into EBs ( Fig. 5b , red dots). Thus, Usp16 is required for the proper regulation of gene expression during ESC differentiation. 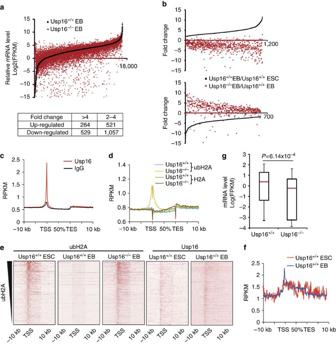Figure 5: Usp16 is required for resolving ubH2A marks during ESC differentiation. (a) Scatter plot of gene expression levels in EBs formed by Usp16+/+(black line) and Usp16−/−ESCs (red dots). mRNA expression level was calculated as log2(FPKM). Summary of genes up- or downregulated in Usp16−/−ESCs was shown in the table. (b) Scatter plot of up- (top panel) and downregulated (bottom panel) genes during Usp16+/+ESC differentiation (black line) as compared with their expression during Usp16−/−ESC differentiation (red dots). Genes were sorted according to log2 fold change in expression. (c) Binding of Usp16 (red line) and IgG (black line) to gene transcribing regions plus 10 kb upstream of TSS and downstream of TES in Usp16+/+EBs. Parallel experiments with Usp16−/−EBs were shown inSupplementary Fig. 5d. (d) ubH2A signal (orange line, Usp16−/−EBs; blue line, Usp16+/+EBs) and H2A signal (brown line, Usp16−/−EBs; green line, Usp16+/+EBs) across gene transcribing regions plus 10 kb upstream of TSS and downstream of TES. (e) ubH2A (first three columns) and Usp16 (fourth and fifth columns) distribution at individual genes in Usp16+/+ESCs, Usp16+/+EBs and Usp16−/−EBs. Genes were sorted based on ubH2A binding in Usp16+/+ESCs. Top 1,000 expressed genes were shown. (f) Usp16 signal in Usp16+/+ESCs (red line) and EBs (blue line) of genes as shown ine. (g) A box and whisker plot, as described inFig. 3a, of the relative expression of ubH2A enriched genes in Usp16+/+and USP16−/−EBs.P-values are calculated by the Student’st-test. Top whisker and bar represent 98th percentile of genes. Bottom whisker and bar represent 2nd percentile of genes above zero. Figure 5: Usp16 is required for resolving ubH2A marks during ESC differentiation. ( a ) Scatter plot of gene expression levels in EBs formed by Usp16 +/+ (black line) and Usp16 −/− ESCs (red dots). mRNA expression level was calculated as log 2 (FPKM). Summary of genes up- or downregulated in Usp16 −/− ESCs was shown in the table. ( b ) Scatter plot of up- (top panel) and downregulated (bottom panel) genes during Usp16 +/+ ESC differentiation (black line) as compared with their expression during Usp16 −/− ESC differentiation (red dots). Genes were sorted according to log2 fold change in expression. ( c ) Binding of Usp16 (red line) and IgG (black line) to gene transcribing regions plus 10 kb upstream of TSS and downstream of TES in Usp16 +/+ EBs. Parallel experiments with Usp16 −/− EBs were shown in Supplementary Fig. 5d . ( d ) ubH2A signal (orange line, Usp16 −/− EBs; blue line, Usp16 +/+ EBs) and H2A signal (brown line, Usp16 −/− EBs; green line, Usp16 +/+ EBs) across gene transcribing regions plus 10 kb upstream of TSS and downstream of TES. ( e ) ubH2A (first three columns) and Usp16 (fourth and fifth columns) distribution at individual genes in Usp16 +/+ ESCs, Usp16 +/+ EBs and Usp16 −/− EBs. Genes were sorted based on ubH2A binding in Usp16 +/+ ESCs. Top 1,000 expressed genes were shown. ( f ) Usp16 signal in Usp16 +/+ ESCs (red line) and EBs (blue line) of genes as shown in e . ( g ) A box and whisker plot, as described in Fig. 3a , of the relative expression of ubH2A enriched genes in Usp16 +/+ and USP16 −/− EBs. P -values are calculated by the Student’s t -test. Top whisker and bar represent 98th percentile of genes. Bottom whisker and bar represent 2nd percentile of genes above zero. Full size image Since severe defects in differentiation were observed in Usp16 −/− EBs, we investigated how Usp16 regulates ESC differentiation by measuring Usp16 binding in Usp16 +/+ EBs and comparing it to the Usp16-binding profile in Usp16 +/+ ESCs. Usp16 binding in both EBs and ESCs is significantly enriched at promoter regions ( Fig. 5c , compare with Fig. 3b ). Parallel experiments in Usp16 −/− EBs did not detect any significant Usp16 binding ( Supplementary Fig. 5c ), confirming the specificity of the ChIP-seq results. About 40% of Usp16-bound promoters in EBs overlap with promoters bound by Usp16 in ESCs ( Supplementary Fig. 5e ). Interestingly, 4,481 genes, which were not bound by Usp16 in ESCs were bound by Usp16 in EBs ( Supplementary Fig. 5e ). These newly bound genes are enriched for transcription regulation, embryonic development, various developmental processes, regulation of biosynthetic process and regulation of macromolecule biosynthetic process ( Supplementary Fig. 5f ). These data indicate that Usp16 might be dynamically recruited to novel targets to regulate ubH2A levels and gene expression during ESC differentiation. Importantly, many of these genes are activated during ESC differentiation. To determine the importance of ubH2A in ESC differentiation, we performed ChIP-seq analysis of ubH2A in Usp16 +/+ and Usp16 −/− EBs. Consistent with the western blot results, we found that ubH2A levels at TSS are significantly increased in Usp16 −/− EBs compared with Usp16 +/+ EBs ( Fig. 5d ). Interestingly, only 57 TSS are significantly enriched for ubH2A in Usp16 +/+ EBs, while 3,100 TSS are enriched for ubH2A in Usp16 −/− EBs ( Fig. 5d ). This demonstrates that Usp16 is required for global H2A deubiquitination during ESC differentiation. The low levels of ubH2A in Usp16 +/+ EBs may indicate that cells in EBs are actively undergoing cell fate transition and, therefore, not many genes are repressed. Parallel experiments with H2A antibody reveal the specificity of the ubH2A ChIP-seq ( Supplementary Fig. 5d ). During ESCs differentiation, ubH2A marks were largely removed ( Fig. 5e ; genes were sorted based on ubH2A level in Usp16 +/+ ESCs). Deubiquitination of ubH2A is strongly linked to Usp16 binding ( Fig. 5e ). Importantly, Usp16-bound genes remain enriched for ubH2A in Usp16 −/− EBs ( Fig. 5e ). Direct comparison of Usp16 binding within these genes revealed that there is a clear increase of Usp16 binding in EBs as compared with ESCs ( Fig. 5e ; quantified in Fig. 5f ). The aberrant enrichment of ubH2A in Usp16 −/− EBs correlated with decreased expression of these genes as compared with Usp16 +/+ EBs ( Fig. 5g ). These data suggest that Usp16 is required to remove the ubH2A repressive marks at developmental genes during ESC differentiation. To confirm our ChIP-seq results, we performed conventional ChIP. As shown in Supplementary Fig. 6 , Usp16 binding to promoter regions of Tbx3, HoxD11 and Gsn genes, which are activated during Usp16 +/+ ESC differentiation, were significantly reduced in Usp16 −/− EBs as compared with Usp16 +/+ EBs. Importantly, the absence of Usp16 binding in Usp16 −/− EBs correlated with increased ubH2A levels at promoter regions. These results suggest that Usp16 is required to resolve the ubH2A repressive marks at developmental genes during ESC differentiation. The primary cause for the differentiation defect of Usp16 −/− ESCs Our studies reveal that Usp16 −/− ESCs do not activate lineage-specific genes and repress pluripotency genes when induced to differentiate ( Figs 4 and 5 ). To determine the primary cause for the undifferentiated phenotype of Usp16 −/− EBs, we tested whether knockdown of pluripotent genes or overexpression of lineage-specific genes could rescue this phenotype. Since EB formation requires prolonged culture and selection of infected cells caused substantial cell death during EB formation, we tested whether the undifferentiated phenotype of Usp16 −/− ESCs could be recapitulated in other culturing systems. For this purpose, we cultured control and Usp16 −/− ESCs in gelatin-coated plates without LIF to induce ESC differentiation. As shown in Fig. 6a,b , when cultured for 6–8 days, control Usp16 +/+ ESCs successfully differentiated, as evidenced by the repression of pluripotent genes Oct4 and Nanog, and activation of lineage-specific genes including Gata4, Gata6 and Hoxc6 (control Usp16 +/+ ). In this culture system, Usp16 −/− ESCs also failed to differentiate, as evidenced by the high expression of Oct4 and Nanog, and low levels of expression of differentiation-associated genes including Gata4, Gata6, Hoxc6, and so on ( Fig. 6a,b ). We next tested whether knockdown of Oct4 could rescue the undifferentiated phenotypes. As shown in Fig. 6a , when Oct4 was significantly knocked down in Usp16 −/− ESCs, Nanog remains highly expressed and lineage-associated genes Gata4, Gata6, Igfbp5 and Hoxc6 remain silenced in these cells (compare Usp16 +/+ and Usp16 −/− with Oct4 KD). These data indicate that the failure to repress pluripotent gene expression is unlikely the primary cause for the undifferentiated phenotype of Usp16 −/− ESCs. 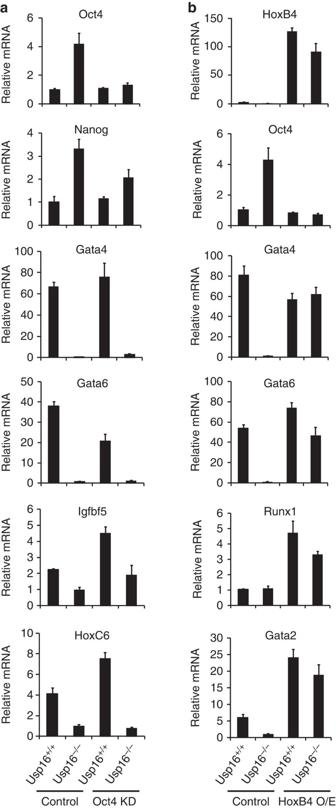Figure 6: The failure to activate lineage-specific gene expression is the cause of undifferentiated phenotype of Usp16−/−ESCs. (a) Knockdown of Oct4 has no effect on Usp16−/−ESC differentiation. RT–qPCR analysis of genes in differentiated Usp16+/+and Usp16−/−ESCs with or without infection of shRNA against Oct4. Bars shown represent means+s.d. Number of biological replicatesn=2. (b) Expression of HoxB4 triggers Usp16−/−ESC differentiation. RT–qPCR analysis of genes in differentiated control and Usp16−/−ESCs with or without infection of HoxB4 lentivirus. Bars shown represent means+s.d. Number of biological replicatesn=2. Figure 6: The failure to activate lineage-specific gene expression is the cause of undifferentiated phenotype of Usp16 −/− ESCs. ( a ) Knockdown of Oct4 has no effect on Usp16 −/− ESC differentiation. RT–qPCR analysis of genes in differentiated Usp16 +/+ and Usp16 −/− ESCs with or without infection of shRNA against Oct4. Bars shown represent means+s.d. Number of biological replicates n =2. ( b ) Expression of HoxB4 triggers Usp16 −/− ESC differentiation. RT–qPCR analysis of genes in differentiated control and Usp16 −/− ESCs with or without infection of HoxB4 lentivirus. Bars shown represent means+s.d. Number of biological replicates n =2. Full size image To determine whether the failure to activate lineage-specific gene expression is the primary cause for the undifferentiated phenotype of Usp16 −/− ESCs, we tested whether the ectopic overexpression of Usp16 target genes, which overcome the repressive ubH2A chromatin marks in Usp16 −/− ESCs, could rescue the undifferentiated phenotype. For this purpose, we expressed Usp16 target gene, HoxB4, in control wild-type Usp16 +/+ and Usp16 −/− ESCs by lentiviral infection. As shown in Fig. 6b , HoxB4 is highly expressed in differentiated Usp16 +/+ and Usp16 −/− ESCs when compared with the uninfected ESCs. Although the expression level of HoxB4 in Usp16 −/− ESCs is slightly lower than in Usp16 +/+ ESCs, pluripotent gene Oct4 was significantly repressed ( Fig. 6b ) and differentiation-associated genes Gata4, Gata6, Runx1 and Gata2 were significantly activated in HoxB4-infected Usp16 −/− ESCs ( Fig. 6b ). These data suggest that the inability to activate lineage-specific gene expression, but not the failure to repress pluripotent genes, is the primary cause for the undifferentiated phenotype of Usp16 −/− EBs. Wild-type Usp16 rescues Usp16 −/− ESC differentiation defect To determine whether defects in Usp16 −/− EB differentiation are due to Usp16 deubiquitinase activity, we electroporated wild type and catalytically inactive Usp16 targeting vectors into Usp16 −/− ESCs. As shown in Fig. 7a , wild-type and mutant Usp16 were expressed at levels similar to that in Usp16 +/− ESCs. Expression of wild-type but not enzymatically inactive mutant Usp16 decreased the ubH2A level in Usp16 −/− ESCs ( Fig. 7a ). When these ESCs were used for EB formation, we found that a significant number of EBs formed from Usp16 −/− ESCs rescued with wild-type Usp16 displayed a differentiated phenotype ( Fig. 7b ; see insertion for relative ratio of differentiated EBs) while virtually all EBs formed from ESCs rescued by catalytically inactive Usp16 exhibited an undifferentiated phenotype ( Fig. 7b ). The differentiated phenotype was further confirmed by RT–qPCR analysis of lineage-specific genes in these EBs. As shown in Fig. 7c , expression of the Igf2, Vimentin, Gata4, Gata6 and Foxa2 genes was significantly increased in EBs formed from Usp16 −/− ESCs rescued by wild-type Usp16. Surprisingly, although there was a modest reduction in the expression of pluripotent genes Oct4 and Nanog, we did not observe a difference between EBs rescued by wild-type or catalytically inactive mutant Usp16 ( Fig. 7c ). This is likely due to the presence of both undifferentiated and differentiated EB populations derived from Usp16 −/− ESCs rescued by wild-type Usp16 ( Fig. 7b ; see insertion for relative ratio of differentiated EB). 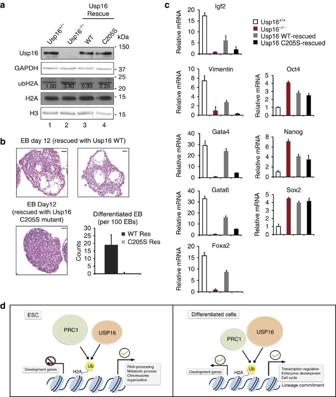Figure 7: Usp16 but not the enzymatically inactive mutant rescues the undifferentiated phenotype of Usp16−/−ESCs. (a) Western blot analysis of Usp16 (top panel) and H2A ubiquitination levels (third panel) in Usp16+/−ESCs, and Usp16−/−ESCs rescued with wild type or enzymatically inactive C205Smutant Usp16. ubH2A signals were quantified as inFig. 2c. Signals in Usp16+/+ESCs were arbitrarily set as 1. GAPDH and histone H3 were used as loading controls. Original scans for blots are shown inSupplementary Fig. 7. (b) Haematoxylin and eosin staining of day12 EBs formed by Usp16−/−ESCs rescued with wild type or enzymatically inactive C205S mutant Usp16. A bar chart summary of EBs exhibiting differentiated phenotype is shown. Scale bar, 100 μm. (c) RT–qPCR analysis of genes in EBs formed by control, Usp16+/−ESCs and Usp16−/−ESCs rescued with wild type or enzymatic inactive C205S mutant Usp16. Bars shown represent means+s.d. Number of biological replicatesn=2. (d) A proposed model for Usp16 and H2A deubiquitination in ESC gene expression and lineage commitment. In ESCs, Usp16 binds to a large number of genes and Usp16 binding inversely correlates with ubH2A levels and positively correlates with gene expression. During ESC differentiation, Usp16 is responsible for reversing H2A ubiquitination at developmental genes, enabling ESC differentiation. Figure 7: Usp16 but not the enzymatically inactive mutant rescues the undifferentiated phenotype of Usp16 −/− ESCs. ( a ) Western blot analysis of Usp16 (top panel) and H2A ubiquitination levels (third panel) in Usp16 +/− ESCs, and Usp16 −/− ESCs rescued with wild type or enzymatically inactive C205Smutant Usp16. ubH2A signals were quantified as in Fig. 2c . Signals in Usp16 +/+ ESCs were arbitrarily set as 1. GAPDH and histone H3 were used as loading controls. Original scans for blots are shown in Supplementary Fig. 7 . ( b ) Haematoxylin and eosin staining of day12 EBs formed by Usp16 −/− ESCs rescued with wild type or enzymatically inactive C205S mutant Usp16. A bar chart summary of EBs exhibiting differentiated phenotype is shown. Scale bar, 100 μm. ( c ) RT–qPCR analysis of genes in EBs formed by control, Usp16 +/− ESCs and Usp16 −/− ESCs rescued with wild type or enzymatic inactive C205S mutant Usp16. Bars shown represent means+s.d. Number of biological replicates n =2. ( d ) A proposed model for Usp16 and H2A deubiquitination in ESC gene expression and lineage commitment. In ESCs, Usp16 binds to a large number of genes and Usp16 binding inversely correlates with ubH2A levels and positively correlates with gene expression. During ESC differentiation, Usp16 is responsible for reversing H2A ubiquitination at developmental genes, enabling ESC differentiation. Full size image Based on these studies, we propose a model for Usp16 in regulating ESC gene expression and differentiation ( Fig. 7d ). In ESCs, Usp16 binds to a large number of genes involved in RNA processing, metabolic process and chromosome organization. The binding of Usp16 is positively correlated with gene expression levels and inversely correlated with ubH2A levels and Ring1B binding. When ESCs are differentiated, Usp16 is required to reverse ubH2A-mediated gene repression and enables gene activation and subsequent ESC differentiation. When Usp16 is absent, the uH2A repressive marks persist at developmental regulators and ESCs do not differentiate. ESCs are valuable resources for regenerative medicine and powerful tools for studying mammalian development. Understanding the molecular mechanisms controlling ESC pluripotency and lineage specification is a prerequisite for its medical application. Epigenetic mechanism plays important roles in establishing and maintaining cell type-specific gene expression programme [2] , [3] , [4] . Previous studies have revealed critical roles for PRC2 and RC1 in repression of lineage-specific gene expression programmes and stabilizing pluripotent gene expression programs in ESCs [3] , [5] , [6] . Previous studies from our laboratory and others reveal that USP16 functions as a histone H2A deubiquitinase to regulate gene expression at specific genes or loci [26] , [43] . However, the genome-binding profile of Usp16 and the genes regulated by Usp16 at a genome scale were not revealed in these studies. Recent studies also reveal that in Down’s syndrome, where Usp16 is triplicated, Usp16 may contribute to somatic stem cell defects [31] . Usp16 has also been shown to coordinate with Aurora B-mediated H3S28 phosphorylation to ensure gene transcription in quiescent lymphocytic cells [32] . Understanding the molecular mechanism of Usp16 is necessary for understanding the function of Usp16 in these processes. In this study, we demonstrated that Usp16 regulates ubH2A levels and gene expression in ESCs. Our data reveal that Usp16 binds to a large number of genes in ESCs, and Usp16 binding is inversely correlated with ubH2A levels and Ring1B binding, and positively correlated with gene expression levels. Usp16 knockout results in a significant increase of ubH2A levels, correlating with a decrease of gene expression. Although Usp16 is not required for ESC viability and self-renewal, Usp16 knockout ESCs have altered gene expression pattern and are not stable at certain culture conditions. Therefore, this study identifies Usp16 and H2A deubiquitination as critical regulators for gene expression to stabilize pluripotent gene expression programme in ESCs. This study adds Usp16 and H2A deubiquitination to the long list of factors regulating ESC function. More significantly, our studies revealed that Usp16 and H2A deubiquitination are required for ESC lineage commitment or differentiation. Usp16 knockout ESCs fail to differentiate. Intriguingly, the failure to activate developmental regulators is the primary cause for the undifferentiated phenotype of Usp16 −/− ESCs. The failure to activate lineage-specific gene expression could be attributed to the inability of Usp16 −/− ESCs to remove repressive ubH2A marks from developmental regulators ( Figs 5 and 6 ). This result highlights the opposing regulatory roles of Usp16-mediated ubH2A deubiquitination to PRC1-mediated ubH2A. Therefore, these studies identify Usp16 and H2A deubiquitination as previously uncharacterized epigenetic mechanisms, which function independently of H3K27me and H3K4me, to control ESC lineage commitment. This study not only provides further evidence for ubH2A in gene silencing [20] , [21] but also a more comprehensive understanding of the functions of H2A ubiquitination in chromatin and cellular regulation. Cell culture Mouse V6.5 (129 × B6 F1 hybrid) ESCs used for gene targeting and C57BL/6J mice for germline transmission are from Dr Tim Townes (University of Alabama at Birmingham). CAGG-Cre mice are from Dr Bradley Yoder (UAB). All derived ESCs were cultured in ESC media, containing DMEM medium (high glucose, Gibco MT-10-013) supplemented with 50 unit per ml penicillin and streptomycin (Life technologies, 15070-063), 18% murine ESC defined FBS (Thermo Scientific, SH30070.03E), 2 mM L -glutamine (Cellgro, 25-005-CI), 1 mM sodium pyruvate (Gibco, 11360-070), 1 × nonessential amino acids (Cellgro, 25-025-CI, 100X stock), 1 × nucleoside (Millipore, ES-008-D, 100 × stock), 0.007% β-mercaptoethanol (Fisher, O3446I) and 1,000 unit per ml mLIF (Millipore, ESGRO) on irradiated mouse embryonic fibroblasts (Millipore, PMEF-NL) and passaged every other day as described previously [16] . For induction of Cre recombinase, Usp16 2lox:2lox :CAGG Cre ESCs were cultured in medium containing 1 μM 4-hydroxytamoxifen (Sigma, H7904) for 3–5 days and then on ESC culture medium. Generation of Usp16 knockout and conditional knockout mice To generate Usp16 knockout and conditional knockout mice, targeting vectors were constructed using sib selection and recombineering technology in DY380 bacteria stain with neomycin selection [44] . Targeting vectors were then electroporated into V6.5 ESCs. After genotyping and sequencing to confirm the correctly recombined knockout allele, Usp16 +/− or Usp16 2lox/+ ESCs were injected into C57BL/6 blastocysts to clone mice. The chimeric mice were backcrossed with C57BL/6 and Usp16 +/− mice were intercrossed for ESC derivation or embryo characterization. Usp16 2lox/+ mice were crossed with CAGG-Cre transgenic mice to obtain Usp16 2lox/+ : CAGG-Cre mice, which was intercrossed or crossed with Usp16 2lox:2lox mice for ESC derivation. Primers used for genotypes are labelled in Fig. 1a and Supplementary Fig. 1a . Primer sequences are included in Supplementary Table 1 . All animal experiments were carried out according to the guidelines for the care and use of laboratory animals of the University of Alabama at Birmingham Institutional Animal Care and Use Committee (IACUC). Derivation and characterization of ESCs Blastocysts were flushed out from the uterus of Usp16 +/− or Usp16 2lox/+ :CAGG-Cre E3.5 female mice with a 27.5 gauge needle connected to 1 ml syringe filled with 1 ml 2i medium [45] . Blastocysts were then transferred to feeder cell plates with 200 μl sterile tip and cultured with 2i medium [46] or regular ESC medium for 5–8 days. ESC-like colonies formed from ICM outgrowths were handpicked using sterile pipette tips and dissociated by 0.25% trypsin and expanded in ESC medium. For proliferation rate assay, 1 × 10 4 ESCs were seeded in 12-well plates and cell numbers were counted and the same seeding procedure was repeated every other day. Western blot assay and qPCR were performed using standard protocol included in the method section [47] . Antibodies include anti-Usp16 (1:1,000) [26] , anti-ubH2A (Millipore, 05–678, 1:1,000), anti-ubH2B (Millipore, 05–1312, 1:1,000), anti-H3 (Abcam, ab100938, 1:5,000), anti-GAPDH (Sigma, G9545, 1:5,000), Anti-Nanog (R&D Systems, AF2729, 1: 2,000), Anti-Oct4 (Santa Cruz Biotechnology, SC9081, 1:2,000) and anti-Sox2 (Cell Signaling, 3579, 1:2,000). Alkaline phosphatase substrate kit was from Vector laboratory (SK-5100). Cell cycle analysis A total of 2 × 10 6 control wild type or Usp16 −/− ESCs were trypsinized and washed with PBS once. Cell pellets were resuspended in 50 μl PBS and 500 μl 0.9% NaCl solution was added to each sample with gentle vortex. 95% ethanol (1.5 ml) was then added to the cell suspension with vortex. Cells were fixed at 4 °C for overnight. After fixation, cells were resuspended in 300 μl PBS with 1 mg ml −1 RNAse (Sigma, R-4875) and incubated at 37 °C for 20 min. Propidium iodide (300 μl, 40 μg ml −1 ; Sigma, P1470) was then added to cell suspension for at least 20 min before proceeding to FACS analysis. EB formation and analysis EBs were formed in EB medium (ESC medium without mLIF) in hanging drops (800 cells per 20 μl drop) on petri dish lids for 48 h. EBs were then collected and cultured on a horizontal rotator at 40 r.p.m. in petri dishes and collected at indicated time points. Medium was changed every other day. For each time point, the diameter of 50 EBs was counted. For H&E staining, EBs were fixed in 4% paraformaldehyde in PBS for 4 h and then in 70% ethanol (overnight), 80% ethanol (1 h), 90% ethanol (1 h), 95% ethanol (overnight), 100% ethanol (1 h, twice), followed by standard H&E staining protocol [47] . Briefly, sample slides were incubated with xylene (5 s, 10 dips), secondary xylene (5 s, 10 dips), 100% ethanol (10 dips), 100% ethanol (3 min), 90% ethanol (3 min), 70% ethanol (3 min), 50% ethanol (3 min), distilled water (3 min), Mayer’s haematoxylin (2 min), running distilled water (20 min), eosin (30 s), 95% ethanol (10 dips), secondary 95% ethanol (10 dips), 100% ethanol (10 dips), 100% ethanol (2 min), xylene (1 min), xylene (2 min) and xylene (3 min). The slides were then covered with cover glass with Permount and dried overnight. RNA purification and real-time PCR assay Total RNA was extracted using TRIzol (Life technologies, 15596-026) following the manufacturer’s instruction. Isolated RNA was reverse transcribed using M-MLV (Promega, M1701) following the manufacturer’s instruction. For quantitative PCR, 0.5 μl cDNA was used as template in a 25 μl reaction containing 1 μg oligo dT 15 primers, 0.5 mM dNTPs, RNase inhibitor, M-MLV and M-MLV buffer. All quantitative PCR reactions were carried out on a Roche LightCycler 480 thermocycler (Roche). Fold change of gene expression levels were calculated according to the 2 −ΔΔ Ct method as described previously [48] and normalized to GAPDH. Primers for real-time PCR assay are listed in Supplementary Table 1 . RNA sequencing and analysis RNA sequencing was performed on Illumina HiSeq2000 in UAB Heflin Genomic Core Facility. cDNA libraries were constructed with TruSeq library generation kits (Illumina). The cDNA ends were repaired, A-tailed and adaptor-ligated for indexing. The cDNA library was then quantified by real-time PCR in a Roche LightCycler 480 with the Kapa Biosystems kit for library quantification (Kapa Biosystems) before cluster generation. Clusters were then generated to yield ~725–825 K clusters per mm 2 and the density and quality were determined after the first base addition. Paired end 2 × 50 bp sequencing runs were performed for all samples. After sequencing, the data was converted to FASTQ Sanger format and then aligned to mouse reference genome mm9 by TopHat [49] . Cufflinks was used to assemble transcripts, estimate the abundances and test for differential expression. Cuffmerge was used to compare the assembled transcripts to the reference annotation across multiple experiments. Cuffdiff was then used to determine the change in transcript levels. Cufflinks, Cuffmerge and Cuffdiff analyses were performed as described previously [50] . Gene ontology analysis was performed using DAVID ( http://david.abcc.ncifcrf.gov/ ). Chromatin immunoprecipitation and ChIP-qPCR assay ESCs were cultured on feeder cell-free plates and fixed with 1% formaldehyde at room temperature for 10 min, followed by quenching with 125 mM glycine. Cells were collected by scraping and washed with PBS once. EBs was dissociated with 0.25% trypsin (Cellgro, MT-25-053-CI) at 37 °C for 10 min before fixation. About 5 × 10 7 cells of ESCs and EBs were resuspended in 10 ml PBS containing 0.5% Triton X-100 and incubated on ice for 10 min. After centrifugation, cell pellets were resuspended in 5 ml Tris-EDTA (TE8.0, pH 8.0) containing 0.1% SDS, and protease inhibitors (0.5 mM pepstatin A, 1 μM leupeptin, 0.5 μM aprotinin and 0.5 mM PMSF). Cell suspension was sonicated using the Fisher sonic dismembrator model 500 at 20% output power 20 times for 30 s followed by a 30-s rest on ice. After sonication, cell suspension was adjusted with 1 × RIPA buffer (10 mM Tris–HCl (pH 8.0), 1 mM EDTA, 0.1% SDS, 0.1% Na-Deoxycholate and 1% Triton X-100) as described previously [51] before immunoprecipitation. About 4–8 μg of affinity-purified Usp16 antibody and an equal amount of IgG were incubated with 150 μl Protein A agarose beads (50% slurry in PBS) at room temperature for 1.5 h and then washed with 1 × RIPA buffer twice to remove unbound antibodies. Antibody–protein A complex was then incubated with 5 ml sonicated chromatin from 5 × 10 7 cells in a 15-ml canonical tube at 4 °C overnight. After incubation, beads were washed in 1.5 ml Eppendorf tubes at 4 °C with 1 ml RIPA buffer (10 min, twice), 1 ml RIPA buffer with 0.3 M NaCl (10 min, twice), 1 ml LiCl buffer (0.25 M LiCl, 0.5% NP40, 0.5% Na-Deoxycholate, 10 min, twice), 1 ml TE 8.0 buffer with 0.2% Triton X-100 (10 min, once) and 1 ml TE 8.0 buffer (10 min, once) [51] . Beads were then resuspended in 100 μl TE 8.0 buffer and crosslinking was reversed by adding 0.5 M NaCl and 1 μg ml −1 RNase A at 65 °C overnight. Additional incubation after adding 3–5 μl of 10% SDS and 5 μl of 20 mg ml −1 protease K was performed at 55 °C for 2 h to fully dissociate protein–antibody complex. DNA template from ChIP was prepared by standard phenol/chloroform DNA extraction and ethanol precipitation. Eluted DNA was dissolved in 50 μl TE 8.0 buffer. For ChIP-qPCR assay, 0.5 μl of 1:5 dilution of elution was used as templates in a 20 μl reactions using GoTag (Promega, M3001) DNA polymerase as described previously [47] . Signals were normalized to input DNA. Primers for ChIP-qPCR are included in Supplementary Table 1 . Native chromatin immunoprecipitation For native ChIP, ESCs and EB (pre-trypsined) were collected and washed with pre-chilled PBS once and incubated in 0.5% NP40 in TBS buffer (10 mM Tris–HCl (pH 7.5), 3 mM CaCl 2 , 2 mM MgCl 2 ) on ice for 1 h with gentle vortex every 15 min. After incubation, cells were homogenized by 10 ml Dounce homogenizer and resuspended in 25% sucrose in TBS. Cells were then transferred to a 15-ml tube prefilled with half volume of 50% sucrose in TBS and spun down at 600 g for 20 min. Pellets were washed in 25% sucrose TBS once and resuspended in nuclear digestion buffer (50 mM Tris–HCl (pH 7.5), 1 mM CaCl 2 , 2 mM MgCl 2 and 0.32 M sucrose) to reach a rough DNA concentration of 0.5 mg ml −1 as measured by Nanodrop. Micrococcal nuclease (MNase; 2 U ml −1 ) was added to the chromatin and digestion was carried out at 37 °C for 15 min and repeated once for the pellet after spinning down the first digestion mixture. Digestion was terminated by addition of 5 mM EDTA. Digested chromatin solution was collected and pellet from second digestion was further incubated with nuclear lysis buffer (1 mM Tris–HCl (pH 7.5), 0.2 EDTA) on ice for 1 h with occasional tapping and then overnight at 4 °C with rotation. The supernatant was collected and combined with the digestion supernatants and stored at −80 °C. All buffers used were supplemented with protease inhibitors, 5 mM PMSF, 5 mM NaF and 2 mM Na 3 VO 4 . For each native ubH2A ChIP, 50 μl beads were incubated with anti-IgM bridging antibody (Millipore, 12–488) for 1 h and washed with 1 ml RIPA buffer containing 0.3 M NaCl. For H2A ChIP, protein G agarose bead was washed with 1 ml RIPA buffer with 0.3 M NaCl. Amount of each antibody used to achieve optimal ChIP performance were determined previously. Briefly, 50 μg ubH2A antibody (Millipore, 05–678) and 15 μg H2A antibody (Millipore, 07–146) were added to treated protein G agarose beads with 400 μg chromatin and incubated at 4 °C for overnight. After immunoprecipitation, beads were washed with 1 ml RIPA buffer (twice, 10 min each), 1 ml LiCl buffer (10 min, once) and 1 ml TE 8.0 (10 min, once). Washed complex were then eluted from beads with 50 mM Tris–HCl (pH 8.0), 1 mM EDTA and 1% SDS by incubation at 65 °C for 5 min and room temperature for 20 min with shaking. Elution process was repeated once and eluates were combined and then incubated at 55 °C for two hours after addition of 5 mM EDTA and 200 μg ml −1 proteinase K. DNA was isolated by phenol–chloroform extraction and ethanol precipitation and dissolved in TE 8.0. ChIP-sequencing and analysis ChIP-sequencing using crosslinked or native chromatin templates was performed at Hudson Alpha Institute Genomic Service Laboratory (GSL) and the National University of Singapore. NEB Next DNA sample prep reagents (New England Biolabs, E6000S/L) were used for end repair, dA-tailing and adaptor ligation (custom adaptors from Hudson Alpha GSL). The entire volume-ligated product was PCR amplified for 15 cycles using Invitrogen’s Pfx DNA polymerase using the custom adaptors designed to allow for 96 unique indexes. Size selection was performed on 2% agarose gel. The final library quality was examined by Qubit and Bioanalysis, and real-time PCR was performed using KAPA’s library quantification kit for Illumina. Each library was diluted to 12.5 pM and clustered using a cBot. Each library was sequenced over 1/6th of a HiSeq 2000 lane following standard Illumina protocols for paired-end 50 bp sequencing. For data analysis, the converted fastq files obtained from Hudson Alpha GSL were aligned to mouse reference genome mm9 by BOWTIE [49] . The SAM files after alignment were filtered to remove PCR duplicate and unmapped reads by SAMtools [52] on Galaxy before converting to Bed files. After Bed files were generated, these files were subjected to peak calling with MACS on Galaxy using an FDR (false discovery rate) threshold set to ≤0.05 (ref. 53 ). Proximal regions around the TSS (−2 kb to +1 kb) that were occupied by at least one peak were defined as enriched promoters/genes. Coordinates of enriched genes with different binding profiles were then intersected to generate Venn diagrams. To count tag density for all the bed files in the coordinates as indicated in all figures, a 15-step workflow on Galaxy ( http://main.g2.bx.psu.edu/ ) was created and available for sharing upon request. To generate heatmaps, individual mm9 gene (RefSeq annotations) was divided into 100 bins using a custom script. Coverage across binned genes plus 10 kb upstream of the TSS and 10 kb downstream of the TES was generated using BEDTools ‘coverageBed’ with the -d option [54] . Outputs were converted to data matrices by a custom script and then visualized as heatmaps in Microsoft Excel 2010 using conditional formatting options. Gene ontology analysis was performed using DAVID ( http://david.abcc.ncifcrf.gov/ ). Usp16 rescue experiment Usp16 −/− ESCs were re-targeted using the same targeting vector or a C205S point mutant vector to generate Usp16 conditional knockout ESCs using procedures similar to those described in the mouse generation method section. Usp16 protein level was measured by western blotting to confirm that wild type or C205S Usp16 was expressed at control levels. EB formation, H&E staining and RT–qPCR assay were performed as described. Oct4 shRNA and HoxB4 overexpression lentivirus infection pLKO-Oc4 shRNA and control vectors were kindly provided by Dr Rui Zhao (UAB Stem Cell Institute). pDL171-HoxB4 and control vectors were kindly provided by Dr Chia-Wei Chang (UAB Stem Cell Institute). Lentiviral vectors together with packaging vectors were transfected in to 293T cell using calcium phosphate and virus were collected at 48 h and 72 h post-infection and pooled. After titration of individual virus, 5 × 10 5 Usp16 −/− ESCs were infected by Oct4 shRNA lentivirus or HoxB4 expression vectors on gelatin-coated six-well plates by spinoculation at room temperature for 2 h and then incubated at 37 °C for overnight before switching to ESC medium. After infection, ESCs were further cultured for 5–7 days before collecting for RNA extraction and RT-qPCR assay. Usp16 +/+ and Usp16 −/− ECS without infection were used as controls. Usp16 and Ring1B overexpression retrovirus infection pMigR1-Usp16 and pMigR1-Ring1B retroviral vectors together with packaging vector were transfected into 293T cells using calcium phosphate and virus were collected at 48 h and 72 h post-infection and pooled. After titration of individual virus, 5 × 10 5 Usp16 +/+ ESCs were infected by Usp16 or Ring1B retrovirus on gelatin-coated six-well plates by spinoculation at room temperature for 2 h and then incubated at 37 °C for overnight before switching to ESC medium. After infection, ESCs were further cultured for 2–3 days before collecting for ChIP–qPCR assay. How to cite this article: Yang, W. et al . The histone H2A deubiquitinase Usp16 regulates embryonic stem cell gene expression and lineage commitment. Nat. Commun. 5:3818 doi: 10.1038/ncomms4818 (2014). Accession numbers The ChIP-Seq and RNA-Seq data for all samples are deposited in the NCBI GEO repository with accession number GSE52899 .